Difluorocarbene enables to access 2-fluoroindoles fromortho-vinylanilines 2-Fluoroindoles as an important structural scaffold are widely existing in many bioactive or therapeutic agents. Despite their potential usefulness, efficient constructions of 2-fluoroindole derivatives are very sparce. The development of straightforward synthetic approaches to access 2-fluoroindoles is highly desirable for studying their fundamental properties and applications. Herein, we report an efficient and general strategy for the construction of 2-fluoroindoles in which a wide variety of 2-fluoroindoles were accessed with high efficiency and chemoselectivity. Instead of starting from indole skeletons, our strategy constructs indole scaffolds alongside the incorporation of fluorine atom on C2 position in a formal [4+1] cyclization from readily accessible ortho -vinylanilines and difluorocarbene. In our protocol, commercially accessible halodifluoroalkylative reagents provide one carbon and one fluorine atom by cleaving one C-N tertiary bond and forming one C-N bond and one C-C double bond with ortho -vinylanilines. Downstream transformations on 2-fluoroindoles lead to various valuable bioactive molecules which demonstrated significant synthetic advantages over previous reports. And mechanistic studies suggest that the reaction undergoes a cascade difluorocarbene-trapping and intramolecular Michael addition reaction followed by C sp 3 -F bond cleavage. The introduction of fluorinated groups (including fluorine atom) into a target molecule would have significant influence on the parent molecule’s reactivity, selectivity, physical and biological properties [1] , [2] , [3] , [4] , [5] , [6] , [7] . Therefore, it becomes a critical strategy in pharmaceuticals for finding therapeutical agents [8] , [9] , [10] , [11] , [12] , [13] , [14] , [15] , [16] , where fluorine atom is often employed as a bioisostere of hydrogen atom based on the above features. Indoles, as one of most important heterocyclic scaffolds, are widespread in a broad variety of natural products [17] , [18] , [19] , [20] and bioactive compounds [17] , [21] , [22] (Fig. 1A , Top). Meanwhile, 2-fluoroindoles are also key structural motifs which are widely existing in some biologically active compounds and demonstrate unique bioactivities [23] , [24] , [25] (Fig. 1A , Bottom). Because of the importance of C2-fluorine-containing indoles in medicinal chemistry, great attention has been devoted to the synthesis of 2-fluoroindoles [26] , [27] , [28] , [29] , [30] , [31] , [32] , [33] , [34] , [35] . However, efficient synthetic methods for the construction of this type of indole derivatives are very rare. Generally, there are three ways to access the target molecules (Fig. 1B ): (a) copper-mediated aminoquinoline-directed fluorination of aromatic C–H bonds. However, there were only 3 examples about 2-fluoroindole synthesis with moderate yields [26] , [27] , and they are limited to 3-aminoquinolineindole derivatives, which seriously limits the application of indole skeleton. (b) pre-functionalization of indoles is mandatory to install some active functional groups, such as –COOH [28] or –SnMe 3 [29] , to C2 position of indoles for further fluorination, which require multi-step synthesis and need toxic organotin reagents, thus severely restrict the substrate scope. (c) silver or base-promoted C–N bond formation from ortho -amino- gem- difluorostyrenes to construct 2-fluororindoles [30] , [31] , [32] , this tactic requires complicated substrates with both gem -difluorostyrene and ortho -aromatic secondary amino functionalities, which are demanding and difficult to access, thus set a severe restriction on their applications in chemical field. Given the paucity of efficient synthetic methods and the huge challenges in the synthesis of 2-fluoroindole derivatives, the development of a convenient approach to synthesize 2-fluoroindole derivatives from simple and readily available starting materials is highly appealing and desirable. Fig. 1: The importance and synthetic approaches to 2-fluoroindoles. A Importance of indoles and 2-fluoroindoles. B Approaches for the construction of 2-fluoroindoles. C Difluorocarbene enables to access 2-fluoroindoles from vinylanilines ( this work ). Full size image Considering the difficulty in accessing the starting materials and limitations of substrates in the previous strategies, we wondered whether a strategy could be developed by using readily accessible starting materials in a one-step protocol. Retrosynthetic analysis of 2-fluoroindole is oriented to the o -alkenylanilines and a reagent which provides both C and F atoms (Fig. 1C ). At this point, halodifluorinated reagents were considered due to their structural motif and their wide applications as fluorinated sources [36] , [37] . In addition, our recent research efforts culminated in discovery and development of several transformations featuring in situ generated difluorocarbene (:CF 2 ) as C1 synthons to assemble various valuable N -containing compounds [38] , [39] , [40] , [41] , [42] , [43] , [44] . Moreover, the intramolecular capture of difluorocarbene by a thiolate and Frustrated Lewis Pairs was also developed [45] , [46] . Therefore, halodifluorinated reagent might be an ideal source to accomplish our goal. Inspired by our pioneering work [38] and the previous research on interaction of tertiary amines with difluorocarbene [47] , [48] , [49] , and considering that difluoromethyl ammonium salt as the key intermediate from tertiary amine is readily decomposed to lead to a difluoromethyl anion in the reaction, we envisage that if a suitable electrophilic group is introduced into the substrate, difluorocarbene can be inserted into the targeted molecule via a nucleophilic attack with both carbon and fluorine atoms on, thus 2-fluoroindole framework might be resulted. There is a challenge in this hypothesis: maintenance of fluorine atom, since fluorine atoms from difluorocarbene are completely discarded and could not be reused in previous reactions, and it is an inevitable shortcoming for such transformations. To our delight, when we installed Michael reaction acceptors (MRAs) [50] , [51] as electrophilic site on the substrates, a series of 2-fluoroindole derivatives were constructed smoothly (>90 examples). This strategy will open an avenue for difluorocarbene-involved transformations and will add significant synthetic values to fluorine chemistry. Herein, we report the first general and highly efficient strategy for the synthesis of 2-fluoroindoles. This method would allow facile entry to construction of 2-fluoroindoles from simple and readily available starting materials under the mild conditions in the absence of transition-metal catalysis, and readily elaborate the late-stage modifications of pharmaceuticals and natural products with broad substrate scope and excellent functional group tolerance, and it will be a groundbreaking synthesis for 2-fluoroindole compounds, which will greatly promote the rapid development of fluorine chemistry and pharmaceutical chemistry [52] , [53] , [54] . Investigation of reaction conditions To validate our conjecture, 3-(2-(dimethylamino)phenyl)-1-phenylprop-2-en-1-one ( 1a ) and BrCF 2 COOEt ( 2a ) were chosen as the model substrates using K 2 CO 3 as base. To our delight, without any other additives in CH 3 CN, the desired 2-flurorindole product 3a was obtained in 76% isolated yield. 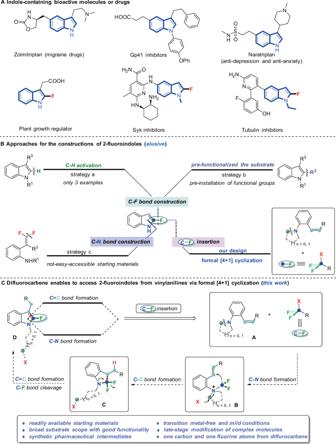Fig. 1: The importance and synthetic approaches to 2-fluoroindoles. AImportance of indoles and 2-fluoroindoles.BApproaches for the construction of 2-fluoroindoles.CDifluorocarbene enables to access 2-fluoroindoles from vinylanilines (this work). Replacing K 2 CO 3 with K 3 PO 4 resulted in a superior result (Table 1 , entry 7), and further base screening indicated that K 3 PO 4 was the best one in comparison with KOH, Cs 2 CO 3 , Na 2 CO 3 , NaOH as well as Na 3 PO 4 (entries 2–7). Encouraged by this promising result, we further screened other solvents (THF, 1,4-dioxane, DME and toluene), and CH 3 CN was found still to be the most effective one (entries 7–11). Difluorinated reagents were subsequently examined and the results suggested that among BrCF 2 COOEt ( 2a ), BrCF 2 PO(OEt) 2 ( 2b ) [55] , TMSCF 2 Br ( 2c ) [56] ClCF 2 COONa ( 2d ), BrCF 2 COOK ( 2e ), BrCF 2 COONa ( 2f ), the best reaction efficiency was endowed by 2a and 2b (entries 12–16). Given the price and the ready accessibility of raw materials, we finally chose 2a as the source of difluorocarbene (See Supplementary Tables 1 – 5 in Supplementary Information for details). Table 1 The condition screening for our difluorocarbene-enabled 2-fluoroindole synthesis. Full size table Synthetic scope With the optimized conditions in hand, we systematically investigated the scope of the difluorocarbene-enabled access to 2-fluoroindoles from ortho -vinylanilines (Fig. 2 ). First, we explored the scope of α,β-unsaturated ketone moiety, which suggested that our reaction was compatible to both aryl and aliphatic α,β-unsaturated ketones. For aromatic ones, substrates bearing electron-neutral ( 1a – 1b ), electron-deficient ( 1c – 1d ), as well as electron-rich substituents ( 1e – 1g ) at the para -position of the aromatic rings all furnished the desired 2-fluoroindole products ( 3a – 3g ) smoothly. And with electronically neutral bis-methyl ( 1h ) and ortho -methyl ( 1i ) substrates, the corresponding products 3h – 3i were procured in 81 and 93% yields respectively. The accommodation of iodine substituents ( 1j ) signified the further potential structural elaborations as a handle. Fused ring reactant like 1-naphthaldehyde ( 1k ) was also a suitable candidate for this transformation. This study was auspiciously and effortlessly extendable to a series of heteroaromatic ketone-containing furan ( 3l ) and thiophene ( 3m ) cores. And for cyclic aryl ketone ( 1o – 1r ), these targeted products could be obtained successfully under the standard conditions as well ( 3o – 3r ). Notably, this protocol also featured an admirable scope with respect to aliphatic ketone substrates. No matter that it was a chain ketone or a cyclic ketone, the corresponding desired products 3s – 3ae were all smoothly delivered (52–80% yields), including four-membered ( 3ab ), six-membered ( 3ac ), eight-membered cyclic ketones ( 3ad ) as well as bicyclic ketone ( 3ae ). Interestingly, substrates tethered with two moieties of reaction sites ( 1n , 1af ) underwent this transformation very well to deliver the products which contain two 2-fluoroindole skeletons ( 3n , 3af ) by simple increasing the equivalent of BrCF 2 COOEt. We next surveyed the scope of R 2 group on the aromatic ring of aniline skeleton. To our delight, a wide range of functionality was compatible under our standard conditions, and alkyl ( 1ag , 1aj ), trifluoromethyl ( 1ah ), alkoxyl ( 1ak ) and halo ( 1ai , 1al – 1an ) substituted substrates were all converted into the corresponding products ( 3ag – 3an ) in moderate to excellent yields (39–81%). To assess the susceptibility of different C–N bonds towards scission, a panel of N -substituted tertiary amines was examined under the standard conditions. 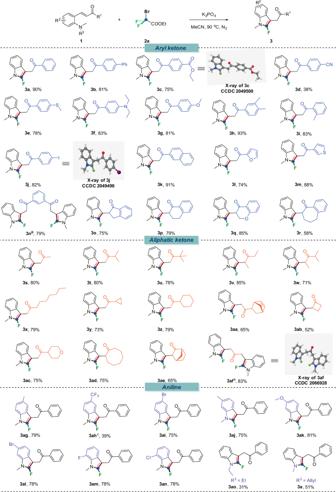Fig. 2: Scope of the α, β-unsaturated ketone-containing anilinesa. Reaction conditions:a1(0.2 mmol),2a(3 equiv., 0.6 mmol), K3PO4(3 equiv.), H2O (0.1 mL), CH3CN (2 mL) under 90 °C for 12 h, N2.b1(0.2 mmol),2a(6 equiv., 1.2 mmol), K3PO4(6 equiv.), H2O (0.15 mL), CH3CN (3 mL) under 90 °C for 12 h, N2.c24 h. N -methylanilines with a different N -substituents ( 1ao , 1ap ) were inspected, and when the R 3 was ethyl group, N -ethylindole ( 3ao ) was obtained in a satisfied yield. Interestingly, when the R 3 is allyl group, contrary to expectations, it was cleaved prior to the C methyl –N bond and 3a was procured in 51% yield. Fig. 2: Scope of the α, β-unsaturated ketone-containing anilines a . Reaction conditions: a 1 (0.2 mmol), 2a (3 equiv., 0.6 mmol), K 3 PO 4 (3 equiv. ), H 2 O (0.1 mL), CH 3 CN (2 mL) under 90 °C for 12 h, N 2 . b 1 (0.2 mmol), 2a (6 equiv., 1.2 mmol), K 3 PO 4 (6 equiv. ), H 2 O (0.15 mL), CH 3 CN (3 mL) under 90 °C for 12 h, N 2 . c 24 h. Full size image We next evaluated the scope of other Michael acceptors (Fig. 3 ), expectedly, these substrates were equipotent to afford the corresponding 2-fluoroindole products in moderate to excellent yields under marginally reoptimized conditions as follows: diethyl BrCF 2 PO(OEt) 2 ( 2b ) as the source of difluorocarbene, K 2 CO 3 as the base and acetonitrile as the solvent at 90 °C for 12 h under N 2 atmosphere (See Supplementary Tables 6 – 7 in Supplementary Information for details). Fig. 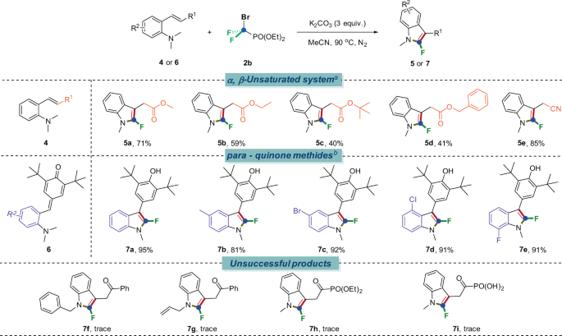Fig. 3: Scope of other α, β-unsaturated system-containing anilines. Reaction conditions:a4(0.2 mmol),2b(3 equiv., 0.6 mmol), K2CO3(3 equiv.), H2O (0.1 mL), CH3CN (2 mL) under 90 °C for 12 h, N2.b6(0.2 mmol),2a(3 equiv., 0.6 mmol), K3PO4(3 equiv.), CH3CN (2 mL) under 90 °C for 12 h, N2. 3: Scope of other α, β-unsaturated system-containing anilines. Reaction conditions: a 4 (0.2 mmol), 2b (3 equiv., 0.6 mmol), K 2 CO 3 (3 equiv. ), H 2 O (0.1 mL), CH 3 CN (2 mL) under 90 °C for 12 h, N 2 . b 6 (0.2 mmol), 2a (3 equiv., 0.6 mmol), K 3 PO 4 (3 equiv. ), CH 3 CN (2 mL) under 90 °C for 12 h, N 2 . Full size image We then first explored α, β -unsaturated esters [50] , [51] . In addition to methyl acrylates, ethyl, tert -butyl and benzyl acrylates were also competent substrates to give the corresponding products ( 5a – 5d ) in moderate yields. Moreover, this system could also enable the synthesis of 2-fluoroindole scaffolds with other Michael acceptors such as acrylonitrile ( 4e ) and para -quinone methides [57] ( 6a – 6e ) with good efficiency, generating functional products ( 5e , 7a – 7e) that are highly valuable structural motifs in medicinal chemistry. In order to further prove the universality of this reaction, we introduced other alkyl groups (like benzyl and allyl group) as substituents on N -atom, and also tried phosphonates (including phosphonic acid) as electron withdrawing groups. However, only trace amount of the corresponding products ( 7f – 7i) was detected. We then tried several other difluoroalkylating reagents which could serve as the sources of difluorocarbene, but no good results were obtained. We also paid our attention to the substrates with different cyclic tertiary amines, if successful, N -tethered long chain aliphatic halides would be rendered, which would add more values for further structural elaborations as a functional handle. The results were summarized in Fig. 4 . It turned out that both four-membered ( 8a ) and five-membered ( 8b – 8u ) cyclic tertiary amines were well-suited for this transformation, exhibiting insensitivity toward aryl substitutions (alkyl, alkoxyl, phenyl, halo, fused, thiophene and furan etc.). The corresponding target products ( 9a – 9u ) were procured in moderate yields. Remarkably, when KI as a nucleophile was added into the reaction system, the N -aliphatic-tethered-iodinated-2-fluoroindoles were obtained ( 9c , 9l , 9p ) in decent yields accordingly. Fig. 4: Scope of cyclic tertiary anilines. Reaction conditions: a 8 (0.2 mmol), 2a (3 equiv., 0.6 mmol), K 3 PO 4 (3 equiv. ), H 2 O (0.1 mL), CH 3 CN (2 mL) under 90 °C for 24 h, N 2 . b 8 (0.2 mmol), 2a (3 equiv., 0.6 mmol), KI (3 equiv. ), K 3 PO 4 (3 equiv. ), H 2 O (0.1 mL), CH 3 CN (2 mL) under 90 °C for 24 h, N 2 . Full size image The above results clearly demonstrated that our method has a broad substrate scope and wide functional group compatibility, which further prompted our endeavors to extrapolate this strategy to late-stage modifications of bioactive molecules and therapeutic agents (Fig. 5 ). Gratifyingly, a series of bioactive molecules (Acetylferrocene, L-valine, DL-proline, Pregnenolone, Adamantane, Progesterone, Geraniol, (-)-Nopol, DL-Menthol, (-)-β-citronellol, Geraniol, Cholesterol) were all derivatized into the corresponding Michael acceptors and installed into our substrates ( 10a – o ) which, upon treatment with BrCF 2 COOEt ( 2a ) or BrCF 2 PO(OEt) 2 ( 2b ) under the established standard conditions, were all smoothly incorporated into the eventual 2-fluoroindole derivatives ( 11a – o ). Moreover, drug compounds, such as (s)-Ibuprofen ( 10m , Antipyretic analgesics), Naproxen ( 10n , Anti-inflammatory), Probenecid ( 10o , Anti-gout agents) were also successfully introduced into the corresponding 2-fluoroindole derivatives ( 11m – o ) without loss of efficiency. By combining the 2-fluoroindole skeleton and bioactive structural motifs together, it was thus envisioned that our system would simplify access to discover more potential bioactive molecules. Fig. 5: Scope of complex molecules a . Reaction conditions: a 10 (0.2 mmol), 2a (3 equiv., 0.6 mmol), K 3 PO 4 (3 equiv. ), H 2 O (0.1 mL), CH 3 CN (2 mL) under 90 °C for 12 h, N 2 . b 10 (0.2 mmol), 2b (3 equiv., 0.6 mmol), K 2 CO 3 (3 equiv. ), CH 3 CN (2 mL) under 90 °C for 12 h, N 2 . Full size image Synthetic application To further demonstrate the synthetic utility of our strategy, we chose 5-chloro- N -methyl-2-fluoroindoles ( 13 ), the key intermediate for the synthesis of Syk (Spleen tyrosine kinase) inhibitors drug, as the target molecule (Fig. 6a ). This reaction could be readily scaled-up from substrate 12a to 5 mmol without loss of efficiency ( 13a , 80% yield). Of note, according to the existing reports [24] , five-step synthesis was required for the construction of 5-chloro- N -methyl-2-fluoroindoles ( 13 ): (1) protection of N-H in indole with tosyl chloride, (2) trimethyltin was installed to activate indole by Sn(Me) 3 Cl, (3) fluorination with selectfluor, (4) removal of sufonamide by KOH, (5) dimethyl sulfate was introduced into the product as a methylation reagent. And for the starting material 12 , it can be obtained by a sequential aromatic nucleophilic substitution between ortho -fluorobenzaldehyes and dimethylamines and aldol condensation between the aforementioned products and ketones. The final product (the starting material 12 for our reaction) could be obtained in the two-step synthesis with a total yield over 90%. And the price of the substrates is very cheap ( ortho -fluorobenzaldehye: 1 $/g, dimethylamine: 0.03 $/g). Compared with the previous method, our route not only significantly decreases the step count (1 step vs. 5 steps), but also could avoid the use of strong base (KOH and NaH), toxic organotin reagents and dimethyl sulfate [58] , [59] . Meanwhile, our strategy could introduce very valuable functional groups in one step on C3 position of indoles as well. HYH42 is a highly specific inhibitor for human non-small cell lung cancer cells (NCI-H460, IC50 < 1 μM) which is commonly used in pharmaceutical research [25] . Remarkably, starting from readily accessible ortho -vinylaniline 15 , our reaction enabled us to access the key intermediate 16 in a single step with a yield of 35% through the direct 2-fluoroindolylation reaction, then HYH42 can be obtained by coupling [25] , [60] from the key intermediate 16 (Fig. 6b ). Moreover, we utilized our methodology on the formal synthesis of 5a , which is the key intermediate of a potential plant growth hormone regulated transcription factor [23] , and the reaction could be scaled up to 5 mmol and the targeted product 5a was obtained in 64% yield (Fig. 6c ). Of note, there is no other efficient report on its synthesis prior to our method. Fig. 6: Synthetic applications. Reaction conditions: a 12 or 15 (0.2 mmol), 2a (3 equiv., 0.6 mmol), K 3 PO 4 (3 equiv. ), H 2 O (0.1 mL), CH 3 CN (2 mL) under 90 °C for 12 h, N 2 . b 12a (5 mmol), 2a (3 equiv., 15 mmol), K 3 PO 4 (3 equiv. ), H 2 O (1.5 mL), CH 3 CN (25 mL) under 90 °C for 24 h, N 2 . c 4a (5 mmol), 2b (3 equiv., 15 mmol), K 2 CO 3 (3 equiv. ), H 2 O (1.5 mL), CH 3 CN (25 mL) under 90 °C for 24 h, N 2 . Full size image Mechanistic studies Intrigued by the features of the presented methodology, we next conducted several control experiments to shed light on the reaction mechanism (Fig. 7 ). When water was replaced by deuterium oxide, one deuterium atom was incorporated at α-position of carbonyl group of the final product 3a-D with 95% deuterization rate in the crude mixture (Fig. 7 , eq. a). When diflurocarbene trapping reagent, namely, benzimidazole ( 18 ), were added individually into this system, 1-(difluoromethyl)-1H-benzo[d]imidazole ( 19 ) was obtained in 78% yield alongside a trace amount of 3a , suggesting the existence of difluorocarbene species (Fig. 7 , eq. b). We then considered whether other dihalocarbene species (:CCl 2 ) are compatible with the reactions, of note, no desired products 20 were detected, which indicates that difluorocarbene species has some special characteristics, which isn’t possessed by other dihalocarbenes (Fig. 7 , eq. c). In order to indicate the essence of tertiary amino group on the substrate, primary amine 21 was subjected to the reaction conditions, not surprisingly, no 2-fluoroindole formation was detected owing to the rapid cyclization to render 2-phenylquinoline 22 (Fig. 7 , eq. d). Moreover, the HRMS (high resolution mass spectrometry) analysis of the mixture of the standard reaction for 30 min showed the two peaks at m/z = 303.1431 and m/z = 288.1199, which matched the ionic compound form possible intermediates 23 and 24 (calcd mass: 303.1429 and 288.1194) (Fig. 7 , eq. e). Fig. 7: Control experiments. a Deuterium-labeling experiment. 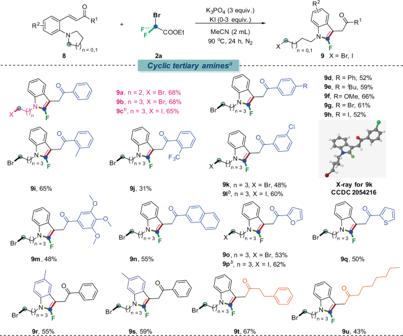Fig. 4: Scope of cyclic tertiary anilines. Reaction conditions:a8(0.2 mmol),2a(3 equiv., 0.6 mmol), K3PO4(3 equiv.), H2O (0.1 mL), CH3CN (2 mL) under 90 °C for 24 h, N2.b8(0.2 mmol),2a(3 equiv., 0.6 mmol), KI (3 equiv.), K3PO4(3 equiv.), H2O (0.1 mL), CH3CN (2 mL) under 90 °C for 24 h, N2. b Diflurocarbene trapping. c Control experiment of dichlorocarbene. d Experiments with non-substituted amino group. e Experiments with HRMS analysis. Full size image Proposed mechanism On the basis of the above results, a plausible mechanism is proposed as depicted in Fig. 8 . Tertiary amine A reacts with the in situ generated difluorocarbene (:CF 2 ) species which is unmasked from halodifluoroalkyl reagents (BrCF 2 COOEt ( 2a ) or BrCF 2 PO(OEt) 2 ( 2b )) in the presence of the base to deliver ammonium salt B . Internal nucleophile (X−) attacks the α carbon of ammonium salt B to break the C–N bond under mild and transition-metal free and oxidant-free conditions [38] , [47] . The newly formed difluoromethyl anion further attacks unsaturated double bond intramolecularly to render intermediate C via Michael addition and protonation. According to our previous work, the CF 2 group on the nitrogen atom is unstable and readily to undertake C–F cleavage under the action of lone pair electrons of the nitrogen atom. Meanwhile, the hydrogen atom adjacent to CF 2 is base-sensitive and easy to be deprotonated, thus a proposed E2cb mechanism is also possible. 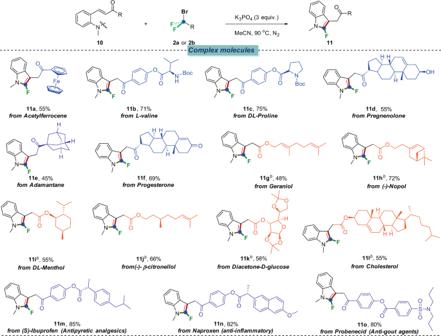Fig. 5: Scope of complex moleculesa. Reaction conditions:a10(0.2 mmol),2a(3 equiv., 0.6 mmol), K3PO4(3 equiv.), H2O (0.1 mL), CH3CN (2 mL) under 90 °C for 12 h, N2.b10(0.2 mmol),2b(3 equiv., 0.6 mmol), K2CO3(3 equiv.), CH3CN (2 mL) under 90 °C for 12 h, N2. Based on the above discussion, there might be two possible paths to render products. One possible path is the C sp 3 –F bond adjacent to N atom is vulnerable in basic conditions to lead to intermediate D via a C sp 3 –F bond cleavage. Finally, with the participation of base, the final product is produced by the driving force to reconstruct the aromatic system (path a). Another way for the formation of the final product is caused by a E2cb pathway with the loss of H-F under basic conditions, once again, the driving force should be the reconstruction of the aromatic ring—indoles (path b). Fig. 8: Plausible mechanism. Possible reaction mechanism of difluorocarbene enables to access 2-fluoroindoles from ortho -vinylanilines. Full size image In summary, we have reported a straightforward synthesis of 2-fluoroindoles from readily accessible ortho -vinylanilines with halodifluoroalkylative reagents as difluorocarbene sources, which provide one carbon atom and one fluorine atom. This general and highly selective transformation provides operationally simple and robust access to versatile 2-fluoroindoles under a mild condition without any transition metals or oxidants. The products obtained can further engage in various derivatizations where the 2-fluoroindole motif functions as an ideal drug skeleton, enabling a fast and orthogonal transformation to many useful building blocks. In a broader context, these features emphasize the value of the presented methodology for the versatile synthesis of 2-fluoroindoles derivatives which are ubiquitously found in bioactive molecules. Further investigations to extend the reaction scope and applications of this process are currently in progress. General procedure for synthesis of 2-fluoroindoles from chalcones or p -Quinone Methide In air, chalcones or p -Quinone Methide (0.2 mmol) and K 3 PO 4 (3 eq, 0.6 mmol) were added to a Schlenk tube equipped with a stir bar. The vessel was evacuated and filled with N 2 (three cycles). BrCF 2 COOEt (3 eq, 0.6 mmol), H 2 O (0.1 mL) and CH 3 CN (2 mL) added in turn by syringe under N 2 atmosphere. The resulting reaction mixture was stirred vigorously at 90 °C for 12 h. Upon completion of the reaction, the solvent was evaporated under reduced pressure and the residue was purified by flash column chromatography to give the desired products. General procedure for synthesis of 2-fluoroindoles from α , β -unsaturated esters or acrylonitrile In air, α, β -unsaturated esters (0.2 mmol) or acrylonitrile and K 2 CO 3 (3 eq, 0.6 mmol) were added to a Schlenk tube equipped with a stir bar. The vessel was evacuated and filled with N 2 (three cycles). BrCF 2 PO(OEt) 2 (3 eq, 0.6 mmol), H 2 O (0.1 mL) and CH 3 CN (2 mL) added in turn by syringe under N 2 atmosphere. 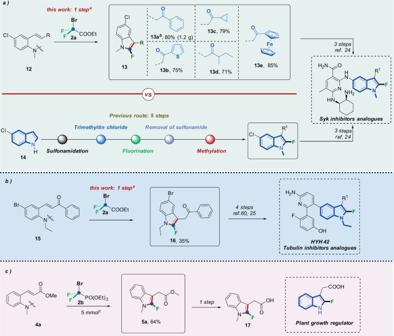Fig. 6: Synthetic applications. Reaction conditions:a12or15(0.2 mmol),2a(3 equiv., 0.6 mmol), K3PO4(3 equiv.), H2O (0.1 mL), CH3CN (2 mL) under 90 °C for 12 h, N2.b12a(5 mmol),2a(3 equiv., 15 mmol), K3PO4(3 equiv.), H2O (1.5 mL), CH3CN (25 mL) under 90 °C for 24 h, N2.c4a(5 mmol),2b(3 equiv., 15 mmol), K2CO3(3 equiv.), H2O (1.5 mL), CH3CN (25 mL) under 90 °C for 24 h, N2. The resulting reaction mixture was stirred vigorously at 90 °C for 12 h. Upon completion of the reaction, the solvent was evaporated under reduced pressure and the residue was purified by flash column chromatography to give the desired products. General procedure for synthesis of N -tethered long chain aliphatic bromine In air, cyclic tertiary amines (0.2 mmol) and K 3 PO 4 (3 eq, 0.6 mmol) were added to a Schlenk tube equipped with a stir bar. The vessel was evacuated and filled with N 2 (three cycles). 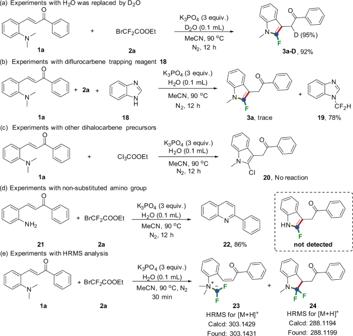Fig. 7: Control experiments. aDeuterium-labeling experiment.bDiflurocarbene trapping.cControl experiment of dichlorocarbene.dExperiments with non-substituted amino group.eExperiments with HRMS analysis. 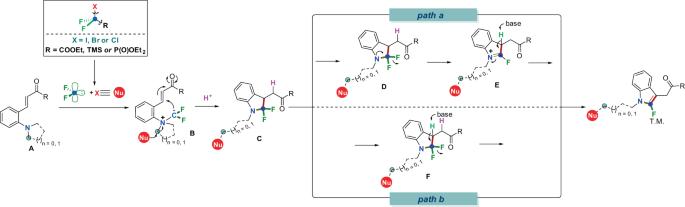Fig. 8: Plausible mechanism. Possible reaction mechanism of difluorocarbene enables to access 2-fluoroindoles fromortho-vinylanilines. BrCF 2 COOEt (3 eq, 0.6 mmol), H 2 O (0.1 mL) and CH 3 CN (2 mL) added in turn by syringe under N 2 atmosphere. The resulting reaction mixture was stirred vigorously at 90 °C for 24 h. Upon completion of the reaction, the solvent was evaporated under reduced pressure and the residue was purified by flash column chromatography to give the desired products. General procedure for synthesis of N -tethered long chain aliphatic iodine In air, cyclic tertiary amines (0.2 mmol), KI (3 eq, 0.2 mmol) and K 3 PO 4 (3 eq, 0.6 mmol) were added to a Schlenk tube equipped with a stir bar. The vessel was evacuated and filled with N 2 (three cycles). BrCF 2 COOEt (3 eq, 0.6 mmol), H 2 O (0.1 mL) and CH 3 CN (2 mL) added in turn by syringe under N 2 atmosphere. The resulting reaction mixture was stirred vigorously at 90 °C for 24 h. Upon completion of the reaction, the solvent was evaporated under reduced pressure and the residue was purified by flash column chromatography to give the desired products.